Low-power nano-optical vortex trapping via plasmonic diabolonanoantennas Optical vortex trapping can allow the capture and manipulation of micro- and nanometre-sized objects such as damageable biological particles or particles with a refractive index lower than the surrounding material. However, the quest for nanometric optical vortex trapping that overcomes the diffraction limit remains. Here we demonstrate the first experimental implementation of low-power nano-optical vortex trapping using plasmonic resonance in gold diabolo nanoantennas. The vortex trapping potential was formed with a minimum at 170 nm from the central local maximum, and allowed polystyrene nanoparticles in water to be trapped strongly at the boundary of the nanoantenna. Furthermore, a large radial trapping stiffness, ~0.69 pN nm −1 W −1 , was measured at the position of the minimum potential, showing good agreement with numerical simulations. This subwavelength-scale nanoantenna system capable of low-power trapping represents a significant step toward versatile, efficient nano-optical manipulations in lab-on-a-chip devices. Fine-scale control of atoms and particles has contributed significantly to addressing key questions in nanoscience [1] , [2] , [3] , [4] . In particular, optical tweezers provide a method to efficiently manipulate micro- and nanometre-sized particles [5] , [6] . The precise control and positioning of dielectric particles using optical trapping techniques can enable promising biomedical applications related to micro-manipulation of cells, bacteria and viruses [7] , [8] . Various optical tweezing technologies for flow cytometry [9] , single-molecule analysis [10] , [11] , photonic force microscopy [12] and optical chromatography [13] were also developed. However, these conventional optical trapping techniques based on free space optics suffer from several drawbacks, such as diffraction-limited trapping volume and significant Brownian motion of the trapped nanoparticles, when the size of trapped particles becomes smaller than light wavelengths [14] , [15] , [16] . Recently, nano-optical trapping techniques based on the use of near-field photonics, such as plasmonic nanoantennas [17] , [18] , [19] , slot waveguides [20] and photonic crystal cavities [21] , have been developed to overcome the limitations imposed by free-space diffraction. In particular, plasmonic nanoantennas, which significantly enhance and confine light in a nano-scale volume [22] , [23] , [24] , allow not only trapping of nano-scale particles smaller than 100 nm [19] , [25] , with relatively low incident power, but also suppression of Brownian motion to the few tens of nanometre scale [17] . Although plasmonic nanoantennas offer a solution to enable subwavelength-scale optical traps, several issues still remain to be addressed. One consideration is that nano-optical potential wells should be formed to possess the shape and depth suitable for a desired application [5] , [26] , [27] , [28] . For example, in biomedical applications using typical plasmonic nanoantennas, particles trapped at the highest intensity region of optical fields could be damaged by absorptive heating, and low-index or absorbing particles feel a repulsive force from the confined optical fields [29] , [30] . Therefore, subwavelength-scale optical vortex trapping is required to capture such damageable biological particles or particles with a refractive index lower than the surrounding material safely and efficiently. In this study, we addressed the quest for miniaturizing optical vortex traps beyond the diffraction limit. By engineering the structure of a plasmonic nanoantenna and adjusting its laser-induced electric field distribution, the nanometric optical vortex trapping potential was formed on the subwavelength-scale landscape. We demonstrated the first experimental implementation of low-power and high-stiffness nano-optical vortex trapping for polystyrene nanoparticles in water and silica nanoparticles in oil via plasmonic gold diabolo nanoantennas, and analysed its unique properties quantitatively using full-field electromagnetic simulations. Diabolo nanoantenna for nano-optical vortex trapping The nano-optical vortex trapping of nanoparticles can be achieved by the plasmonic resonance excited and enhanced along the boundary of the metallic nanoantenna. 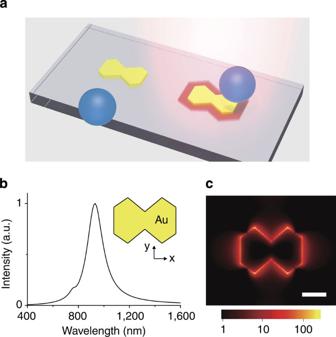Figure 1: Plasmonic diabolo nanoantenna. (a) Schematic diagram of the optical vortex trapping of nanoparticles using a plasmonic diabolo nanoantenna. (b) Calculated spectrum of the electric field intensity enhancement. The inset shows the top-view of the simulated gold diabolo nanoantenna. (c) Calculated electric field distribution (log-scale) excited byx-polarized incident light with a wavelength of 980 nm. The scale bar is 200 nm. Figure 1a shows a schematic diagram of optical vortex trapping using a gold diabolo nanoantenna. By injecting a 980 nm laser, the localized plasmonic resonance is excited in the nanoantenna and produces a nanometric optical potential well to trap a polystyrene particle immersed in water [17] , [18] , [20] , [21] , [25] . A three-dimensional finite-difference time-domain (3D FDTD) simulation was performed to examine the electric field distribution in the diabolo nanoantenna and determine its optimized structural parameters [31] , [32] , [33] . Figure 1b shows that a plasmonic resonance peak appeared at 980 nm in the gold diabolo structure with a thickness of 15 nm and horizontal length of 500 nm on a glass substrate. In this structure, we also calculated the electric field distribution excited by x -polarized incident light with a wavelength of 980 nm ( Fig. 1c ). As all sides of the diabolo nanoantenna are not parallel to the incident polarization direction, the electric fields can be enhanced evenly along the entire boundary of the structure [32] , [34] . Furthermore, 260-fold intensity enhancement was achieved at the electric field maximum compared with the incident light intensity. Such a field distribution is distinguishable from those of conventional metallic nanoantennas yielding field enhancement only at a specific region [17] , [18] , [19] , [23] , [24] . The unique near-field distribution of the diabolo nanoantenna can cause a strong optical gradient force and the nano-optical vortex trapping of nanoparticles. Figure 1: Plasmonic diabolo nanoantenna. ( a ) Schematic diagram of the optical vortex trapping of nanoparticles using a plasmonic diabolo nanoantenna. ( b ) Calculated spectrum of the electric field intensity enhancement. The inset shows the top-view of the simulated gold diabolo nanoantenna. ( c ) Calculated electric field distribution (log-scale) excited by x -polarized incident light with a wavelength of 980 nm. The scale bar is 200 nm. 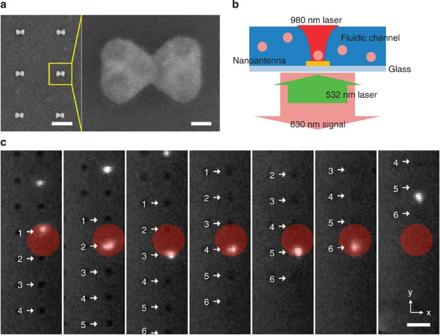Figure 2: Optical trapping of polystyrene nanoparticles via diabolo nanoantenna array. (a) Scanning electron microscopy image of the fabricated gold diabolo nanoantenna array (left) and magnified image of a single nanoantenna (right). The scale bars are 1 μm (left) and 100 nm (right). (b) Schematic diagram of the optical trapping measurement setup. Two lasers with wavelengths of 980 and 532 nm were used for the optical trapping and excitation of fluorescence of the particles, respectively. The particles emitted fluorescence with a centre wavelength of ~630 nm. (c) Successive charge-coupled device images of the trapped particles. The nanoantennas moved along theyaxis with the position of the 980 nm laser fixed (red circle). The white arrows indicate the positions of the nanoantennas. The scale bar is 2 μm. Full size image Nanoantenna trapping experiments The fabricated gold diabolo nanoantennas are shown in the scanning electron microscopy images of Figure 2a . The 15 nm thick gold structures were fabricated on a glass cover slip using a conventional lift-off process (Methods) [24] . The actual intensity enhancement factor in the fabricated nanoantenna could be reduced to ~85. The nanoantennas were placed in a fluidic chamber with deionized water containing 300-nm-diameter fluorescent polystyrene particles. A continuous-wave 980 nm laser diode with a power of ~5.5 mW was used to excite the plasmonic resonance for optical trapping ( Fig. 2b ). A ×40 microscope objective lens was used to focus this laser beam to the full-width at half-maximum (FWHM) of ~1.4 μm. The optical potential well and trapping force were then generated efficiently around the nanoantenna. In addition, the fluorescent polystyrene particles were excited by a laser with a wavelength of 532 nm and power of 300 nW μm −2 through the glass substrate ( Fig. 2b ). The fluorescence from the particles passing through a 630 nm band-pass filter was measured using an electron multiplying charge-coupled device (EMCCD) camera, which can indicate the positions of these particles accurately [18] , [20] , [21] . We note that this 532 nm laser was too weak to affect the trapping process. Figure 2: Optical trapping of polystyrene nanoparticles via diabolo nanoantenna array. ( a ) Scanning electron microscopy image of the fabricated gold diabolo nanoantenna array (left) and magnified image of a single nanoantenna (right). The scale bars are 1 μm (left) and 100 nm (right). ( b ) Schematic diagram of the optical trapping measurement setup. Two lasers with wavelengths of 980 and 532 nm were used for the optical trapping and excitation of fluorescence of the particles, respectively. The particles emitted fluorescence with a centre wavelength of ~630 nm. ( c ) Successive charge-coupled device images of the trapped particles. The nanoantennas moved along the y axis with the position of the 980 nm laser fixed (red circle). The white arrows indicate the positions of the nanoantennas. The scale bar is 2 μm. Full size image The trapping experiment was performed in an array of nanoantennas with a period of 2 μm ( Fig. 2c ). To examine the optical trapping of the particles, the substrate including the nanoantennas was placed on an x-y translation stage and moved along the y axis with the position of the 980 nm laser fixed. In Figure 2c , each position of the laser is marked by a red circle with a diameter of two times the FWHM of the laser spot. Indeed, the measurement showed that the polystyrene particles emitting fluorescence were trapped strongly only at the regions of the nanoantennas. The particles moved in a step-like manner from one illuminated nanoantenna to the next as the nanoantenna array moved (see also Supplementary Movie 1 ) [17] . In particular, the particle was successfully trapped, even though the nanoantenna was located at the edge of the laser spot and the incident laser power on the nanoantenna was relatively low. On the other hand, optical trapping was not achieved by the 980 nm laser itself without the nanoantenna because the trapping potential well was not deep enough to overcome the kinetic energy of Brownian motion at room temperature (the right most panel, Fig. 2c ) [6] , [14] . This indicates that the motions of trapped particles were determined dominantly by the strongly enhanced near-fields of the nanoantennas. Position tracking of a single trapped particle The measured distribution of the position of a single polystyrene particle trapped on a nanoantenna was plotted to examine the optical vortex trapping ( Fig. 3a ). The motion of the particle was captured by EMCCD during 80 s with a camera speed of 30 Hz ( Supplementary Movie 2 ), and the centroid algorithm was then used to determine the centre position of the particle [6] . The spatial resolution of the particle position obtained in this experimental system was ~5.5 nm, which was much higher than the resolution determined by the pixel size of the EMCCD, ~150 nm, and the diffraction limit of the objective lens used in the measurement setup. As shown in a representative distribution of the particle position ( Fig. 3a ), the particle was trapped tightly around the boundary of the diabolo nanoantenna where strong field enhancement was achieved by the plasmonic resonance. We underscore that this nano-optical vortex trapping of a small particle with a diameter of 300 nm was successfully demonstrated with a low power of ~5.5 mW. 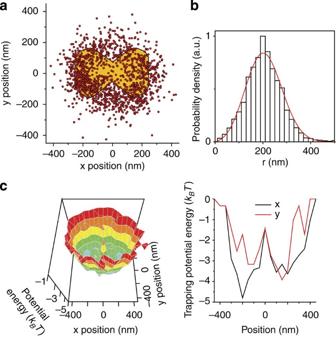Figure 3: Measurement of optical vortex trapping of a single particle. (a) The measured position distribution of a trapped single polystyrene particle. The fabricated diabolo nanoantenna was superimposed on it. (b) The histogram of the probability density plotted as a function of the distance from the centre of nanoantenna to the particle position,r. The data is from (a). The red line is a fit to the histogram with the Boltzmann probability density function to estimate the radial trapping stiffness and the position of minimum potential energy. (c) The trapping potential energy obtained from the trapping position distribution of (a). The 3D plot of the trapping potential energy (left) and its cross-sectional views along thexandyaxes (right) are shown. Figure 3: Measurement of optical vortex trapping of a single particle. ( a ) The measured position distribution of a trapped single polystyrene particle. The fabricated diabolo nanoantenna was superimposed on it. ( b ) The histogram of the probability density plotted as a function of the distance from the centre of nanoantenna to the particle position, r . The data is from ( a ). The red line is a fit to the histogram with the Boltzmann probability density function to estimate the radial trapping stiffness and the position of minimum potential energy. ( c ) The trapping potential energy obtained from the trapping position distribution of ( a ). The 3D plot of the trapping potential energy (left) and its cross-sectional views along the x and y axes (right) are shown. Full size image The doughnut-shaped vortex trapping was also observed in the histogram of the probability density, which was plotted as a function of the distance from the centre of nanoantenna to the particle position, r ( Fig. 3b ). The highest probability density was obtained at r ~ 200 nm, not at the centre. We note that the position of the highest probability density does not faithfully reflect that of the minimum potential energy [35] . To calculate the radial trapping stiffness and the position of minimum potential energy in this vortex trapping, we employed the Boltzmann probability density function, where A is the normalization constant satisfying U ( r ) is the trapping potential energy, k B is the Boltzmann constant and T is the temperature [6] , [35] . The potential energy regarded as a parabolic function [35] , was used to fit the probability density (red line, Fig. 3b ), where k r is the radial trapping stiffness and r 0 is the position of minimum potential energy. As a result of this fitting, k r and r 0 were estimated to be 0.69 pN nm −1 W −1 and 170 nm, respectively. The large trapping stiffness, which was normalized by the illuminated power to the physical cross section of the nanoantenna, is comparable to those of previously reported nano-optical tweezers using slot waveguides [20] , photonic crystal cavities [21] or plasmonic structures [17] , [25] , [27] . In addition, the small value of r 0 is indicative of a miniaturized nano-optical vortex trap overcoming the diffraction limit. Therefore, our subwavelength-scale nanoantenna system can offer the capability to strongly trap a small particle with low incident power. To assess the trapping potential energy as a function of the position, the distribution of the particle position of Figure 3a was examined. The potential energy distribution in the x−y plane can be calculated directly using the Boltzmann probability distribution function [6] . Figure 3c shows the 3D plot of the potential energy obtained from the distribution of Figure 3a as a function of the x and y positions, where the spatial resolution of the trapping potential was 50 nm. The minima of the potential energy appeared at the position <200 nm away from the centre of the nanoantenna, whereas the local maximum was at the centre. This result shows the proper formation of the optical vortex potential well to trap particles at the boundary of the nanoantenna [5] , [26] , [29] , [30] . Additionally, as shown in the cross-sectional views of the trapping potential energy in the x and y axes ( Fig. 3c ), the depth of the potential energy was large enough to trap the particle, compared with the kinetic energy of Brownian motion at room temperature, k B T [6] , [14] . Trapping force simulation To further understand the experimental results, we calculated the trapping force using 3D FDTD simulation ( Fig. 4 ). The Maxwell's stress tensor was solved directly to calculate the sum of the forces on the entire surface of the polystyrene particle (Methods) [20] , [21] , [36] . In the simulation, the polystyrene particle is a dielectric sphere with a diameter of 300 nm and a refractive index of 1.57, and its centre is 165 nm distant from the top surface of the gold nanoantenna in the vertical direction. 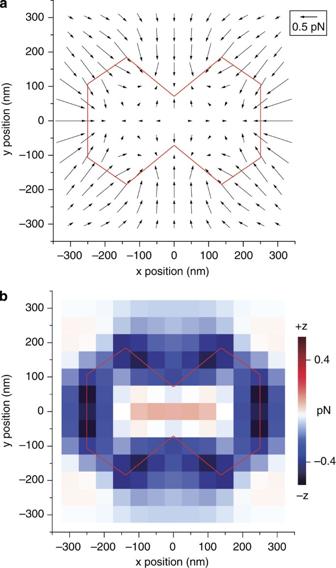Figure 4: Calculated horizontal and vertical components of optical force acting on a polystyrene particle. (a) Calculated horizontal component of the optical force in the x-y plane as a function of the x and y positions of the particle centre. The scale bar is 0.5 pN. The centre of the particle was assumed to be 165 nm distant from the top surface of the nanoantenna in the simulation. (b) Calculated vertical (zaxis) component of the optical force as a function of thexandypositions of the particle centre. The negative and positive optical forces indicate the attractive and repulsive ones to the nanoantenna, respectively. In (a) and (b), the diameter of the polystyrene particle was 300 nm. By injecting the plane wave with a wavelength of 980 nm and power density of 6.1 mW μm −2 , which is similar to the experimental condition, the horizontal ( F x and F y ) and vertical ( F z ) components of the optical force acting on the particle were calculated and plotted as a function of the x and y positions of the particle centre in Figure 4a,b , respectively. Both horizontal and vertical components indeed force the particle to move to the boundary of the nanoantenna with maximum electric near-fields. Therefore, this simulation result shows that the 3D optical vortex trapping of a particle can be achieved faithfully and also provides an excellent reproduction of the experimental results in Figures 2c and 3a . In addition, the optical force and trapping stiffness were calculated under similar conditions to the experiment. The maximum horizontal and vertical optical forces, ~1.0 pN and ~0.58 pN, respectively, were obtained near both horizontal ends of the nanoantenna. Furthermore, a trapping stiffness was calculated using the slope of the optical force variation [6] , [20] , [21] . A large trapping stiffness of ~0.34 pN nm −1 W −1 was calculated at the position of the deepest potential energy in the x axis, showing good agreement with the measured stiffness. Figure 4: Calculated horizontal and vertical components of optical force acting on a polystyrene particle. ( a ) Calculated horizontal component of the optical force in the x-y plane as a function of the x and y positions of the particle centre. The scale bar is 0.5 pN. The centre of the particle was assumed to be 165 nm distant from the top surface of the nanoantenna in the simulation. ( b ) Calculated vertical ( z axis) component of the optical force as a function of the x and y positions of the particle centre. The negative and positive optical forces indicate the attractive and repulsive ones to the nanoantenna, respectively. In ( a ) and ( b ), the diameter of the polystyrene particle was 300 nm. Full size image Trapping of a single silica particle in oil To take full advantage of nano-optical vortex trapping, we performed trapping experiments using silica nanoparticles immersed in oil ( Fig. 5 ). A continuous-wave 980 nm laser diode with a power of ~23 mW and the FWHM of ~5 μm was used to excite the plasmonic resonance of the nanoantenna. The silica particle was illuminated by tungsten halogen lamp, and the scattered light from the particle was measured using an EMCCD camera with a speed of 30 Hz during 10 s (Methods). The centroid algorithm was also used to determine the centre position of the single silica particle [6] . 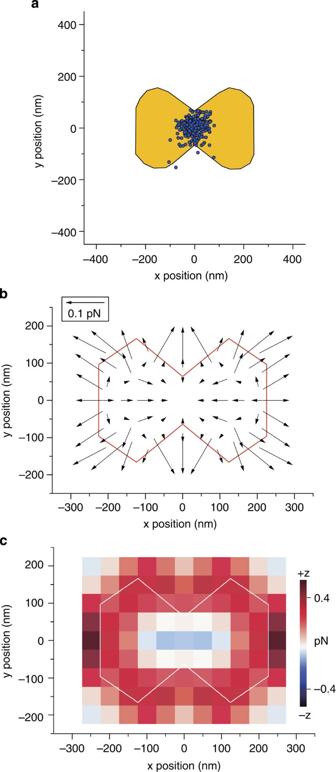Figure 5: Nano-optical vortex trapping of a single silica particle in oil. (a) The measured position distribution of a trapped single silica particle in oil. The diameter of the silica particle is 300 nm, and the refractive indices of the silica particle and oil are 1.45 and 1.62, respectively. (b) Calculated horizontal component of the optical force in thex-yplane as a function of thexandypositions of the particle centre. The scale bar is 0.1 pN. The horizontal length of the nanoantenna is 450 nm and the centre of the particle is 165 nm distant from the top surface of the nanoantenna in the simulation. The plane wave with a wavelength of 980 nm and power density of 6.1 mW μm−2is injected. (c) Calculated vertical (zaxis) component of the optical force as a function of thexandypositions of the particle centre. In Figure 5a , the measured position distribution of the particle shows that the silica particle was trapped tightly at the centre of the diabolo nanoantenna with a local minimum of electric field intensity while the gradient force repels the silica particle from the high intensity region around the boundary of the nanoantenna [29] . This is distinguishable from the result of Figure 3a because the refractive index of the silica particle, 1.45, is lower than that of oil, 1.62. In addition, we note that the FDTD simulations of Figure 5b,c agree well with the experimental result of Figure 5a . This result shows the successful demonstration of nano-optical vortex trapping using particles with a refractive index lower than the surrounding material. Figure 5: Nano-optical vortex trapping of a single silica particle in oil. ( a ) The measured position distribution of a trapped single silica particle in oil. The diameter of the silica particle is 300 nm, and the refractive indices of the silica particle and oil are 1.45 and 1.62, respectively. ( b ) Calculated horizontal component of the optical force in the x-y plane as a function of the x and y positions of the particle centre. The scale bar is 0.1 pN. The horizontal length of the nanoantenna is 450 nm and the centre of the particle is 165 nm distant from the top surface of the nanoantenna in the simulation. The plane wave with a wavelength of 980 nm and power density of 6.1 mW μm −2 is injected. ( c ) Calculated vertical ( z axis) component of the optical force as a function of the x and y positions of the particle centre. Full size image We successfully demonstrated a nanometric optical vortex trap via plasmonic diabolo nanoantennas for the first time. The optical vortex potential energy, which was formed by plasmonic resonance in the metallic nanoantenna, allowed the strong trapping of polystyrene nanoparticles in water around the boundary of the nanoantenna, whereas the silica nanoparticles in oil were trapped tightly at the centre. The large optical force and trapping stiffness achieved in our subwavelength-scale nanoantenna system can offer the capability to trap nanoparticles with low power and therefore will be highly useful for biomedical applications that require reduced heating and damage in biological particles [18] , [20] , [37] . Fabrication of the nanoantennas The gold nanoantennas were fabricated using the following processes. Electron-beam lithography was performed at an acceleration voltage of 30 keV on a 150-μm thick glass cover slip. The 0.3 nm thick chromium adhesion layer and 15 nm thick gold layer were then deposited using an electron-beam evaporator at a deposition rate of 0.3 Å s −1 , and a lift-off process with acetone was followed. Experimental setup The glass cover slip with nanoantennas was attached to a slide glass using 50 μm thick double side sticky tape. A 50 μm thick fluidic channel was then formed between the cover slip and slide glass. Two holes for the inlet and outlet of the fluidic chamber were drilled in the slide glass. Deionized water with 2% of polysorbate 20 (Tween 20) containing the fluorescent polystyrene particles with diameters of 300 nm (Thermo Scientific Inc.) was injected into the fluidic chamber through a syringe and syringe pump, and a 532 nm laser was used to excite the fluorescent polystyrene particles with a centre fluorescence wavelength of ~630 nm ( Figs 2 and 3 ). Oil with a refractive index of 1.62 (Cargille Labs, refractive index liquids series A) containing the silica particles with diameters of 300 nm (Microspheres-Nanospheres company) was used for trapping experiments in Figure 5 , where the silica particles were illuminated by a tungsten halogen lamp. A ×100 oil immersed objective lens was used to collect either the fluorescence from the polystyrene particles ( Figs 2 and 3 ) or the scattered light from the silica particles ( Fig. 5 ) through the cover slip. In addition, a 980 nm laser was injected from the slide glass to excite the plasmonic resonance in the nanoantenna. FDTD simulations In the 3D FDTD simulation ( Figs 1b,c , 4 and 5b,c ), the metal was modelled with the dielectric function of the free electron gas (Drude model): ɛ ( ω )= ɛ ∞ − ω p 2 /( ω 2 + iγω ). The Drude model was used to fit the experimentally determined dielectric function of gold in the spectral range from 600 to 1,400 nm. The background dielectric constant ɛ ∞ , plasma frequency ω p and collision frequency γ at room temperature were set to 12.99, 1.453×10 16 s −1 and 1.109×10 14 s −1 , respectively [33] . In the calculation of the optical properties of the nanoantenna, the domain size and grid size were 3.0×3.0×2.0 μm 3 and 5.0 nm, respectively. The uniaxial perfectly matched layer was used as the absorbing boundary condition. Optical force calculations The time-averaged optical force on a particle, ‹ F ›, was calculated using the following integral of Maxwell's stress tensor, ( Figs 4 and 5 ): where V and S are the volume and surface containing only the particle, respectively. Maxwell's stress tensor can also be represented by the interaction between electric/magnetic forces and mechanical momentum as follows [36] : The electric/magnetic field distributions obtained by the 3D FDTD simulation were used to calculate Maxwell's stress tensor and the optical force in these equations: we calculated the electric/magnetic field distribution for each location where the force is calculated. How to cite this article: Kang, J.-H. et al . Low-power nano-optical vortex trapping via plasmonic diabolo nanoantenna. Nat. Commun. 2:582 doi: 10.1038/ncomms1592 (2011).